Referential gestures in fish collaborative hunting In humans, referential gestures intentionally draw the attention of a partner to an object of mutual interest, and are considered a key element in language development. Outside humans, referential gestures have only been attributed to great apes and, most recently, ravens. This was interpreted as further evidence for the comparable cognitive abilities of primates and corvids. Here we describe a signal that coral reef fishes, the grouper Plectropomus pessuliferus marisrubri and coral trout Plectropomus leopardus , use to indicate hidden prey to cooperative hunting partners, including giant moray eels Gymnothorax javanicus , Napoleon wrasses Chelinus undulatus and octopuses Octopus cyanea . We provide evidence that the signal possesses the five attributes proposed to infer a referential gesture: it is directed towards an object, mechanically ineffective, directed towards a potential recipient, receives a voluntary response and demonstrates hallmarks of intentionality. Thus, referential gesture use is not restricted to large-brained vertebrates. From infancy humans communicate in complex ways using gestures [1] , which can be defined as intentional signals in that they are targeted at a recipient with the aim of influencing its behaviour in a specific way [2] . Human infants use gestures such as pointing, showing or giving to draw the attention of a social partner to a specific entity in the environment [1] . These signals can be classified as referential based on this function [3] , [4] . Referential signals may be used to share interest in an object or to achieve a more tangible aim such as retrieving the item. Pointing is one of the most widely used human referential gestures [5] . It strongly predicts language development [1] , [6] and has been suggested as a key component of language acquisition [7] . In contrast to evidence of their frequent use by humans, examples of referential gestures by other species are rare. Most examples are from great apes in captivity that gesture referentially to human experimenters [4] , [8] , [9] , [10] . In the wild, chimpanzees seem to use directed scratches to indicate areas of their body they wish to be groomed by conspecifics [11] , and observations suggest that bonobos point to indicate potential threats to conspecifics [12] . Recently, Pika and Bugnyar [13] provided evidence for the use of referential gestures by a non-primate in their study on wild ravens that show and offer non-food items to conspecifics apparently in the context of social bonding between pair partners. Pika and Bugnyar interpreted their results as further evidence that, in some domains, the cognitive abilities of corvids are comparable to those of primates [14] , [15] . Although the cognitive similarities between these two large-brained clades may well hold true with respect to their long list of shared abilities, an ecologically driven concept of cognition would predict that any single capacity may evolve as a function of ecological need [16] , [17] , [18] . A species which may exemplify selection for the ability to gesture referentially is the roving coral grouper Plectropomus pessuliferus marisrubri (hereafter ‘grouper'), which has been observed to use a specific signal to indicate the location of hidden prey to collaborative hunting partners [19] . Groupers regularly hunt collaboratively with other fish species, in particular the giant moray eel Gymnothorax javanicus (hereafter ‘moray'), and also the Napoleon wrasse Cheilinus undulatus (hereafter ‘wrasse') [19] . Partner species benefit from hunting together because of their naturally complementary hunting tactics. The grouper possesses burst speed to capture prey in open water, while morays and wrasses may access prey hiding in reef cracks and crevices. Morays may physically move inside crevices because of their slender body, while wrasses have powerful protractile jaws that can suck out hidden prey or smash the reef matrix around it. When two predators with complementary hunting techniques hunt simultaneously, they may increase their hunting success rate [19] . The grouper has been shown to use two distinct signals to coordinate collaborative hunts. The first and most commonly used is a high frequency shimmy of its entire body, performed while horizontal and in front of a sheltering moray, which typically causes the moray to accompany the grouper in a joint search for potential prey (see video S1 of Bshary et al . [19] ). The moray may not begin joint hunting in response to the grouper’s first shimmy signal and often interrupts the joint hunt by sheltering in the coral. In these cases the grouper will often resignal to the moray multiple times until the moray begins to move, with signals punctuated by short breaks where the grouper will often look towards the moray. This shimmy signal appears to fulfil the criteria for a gesture as defined by Hobaiter and Byrne [2] ; it is a discrete and mechanically ineffective movement of the body that is targeted at a recipient, used to elicit a specific behaviour in the recipient (joint activity in this case), and appears to be used intentionally as indicated by persistence towards the goal of eliciting joint activity. However, this gesture is not referential as it is not used to direct the recipient’s attention towards an external entity; potential prey are encountered opportunistically during the joint hunt. In contrast, the grouper’s second signal, whereby it orientates itself vertically and head-down while conducting distinct headshakes with pauses between them (see video S3 of Bshary et al . [19] ), does appear to indicate an object. Although occurring infrequently, this headstand signal has only been observed over the location of an escaped prey fish after an unsuccessful chase by the grouper. It appears to indicate the location of the hidden prey to hunting partners such as morays and wrasses [19] . The signal thus focuses the attention of both partners on a specific object (the crevice where the prey escaped). Bshary et al . [19] were only concerned with the phenomenon of collaborative hunting between species, and were unaware of the possibility that the grouper’s headstand signal is a referential gesture. Fortunately, Bshary’s observations of grouper collaborative hunting were documented in a descriptive text. In the present study, we reanalyse their data to determine whether the grouper’s headstand qualifies as a referential gesture. On the basis of Pika [20] , Pika and Bugnyar [13] set out attributes that they use to qualify a signal as a referential gesture. On the basis of the attributes described by Pika and Bugnyar [13] we can extract five general criteria for this form of signalling. Namely, the signal must be directed towards a referent, mechanically ineffective for any purpose other than a signal, directed towards a potential recipient, receive a voluntary response and demonstrate hallmarks of intentional production. With respect to the last criterion, numerous behaviours have been used previously as hallmarks of intentional signal production [9] , [20] , [21] . Those we provide are not the same as used by Pika and Bugnyar [13] but are considered by some authors as the key indicators of intentional signal production [21] . By examining our data on headstand signalling between the grouper and its hunting partners with respect to the five criteria, we find that this signal qualifies as a referential gesture. Furthermore, we report for the first time that another Plectropomid species, the coral trout Plectropomus leopardus (hereafter ‘coral trout'), hunts collaboratively and headstand signals in a similar manner to the grouper, but in its case to octopus ( Octopus cyanea , hereafter ‘octopus') hunting partners on the Great Barrier Reef. Our results thus show that referential gestures are not restricted to large-brained species and suggest they may have evolved in other taxa with an ecological need for them. 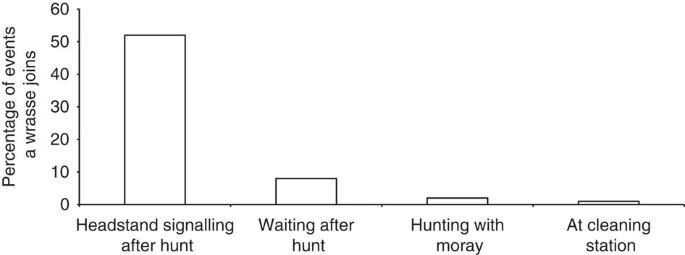Figure 1: Attraction of wrasses to the headstand gesture. The percentage of events in which a wrasse comes within 10 m of the grouper within 5 min of the grouper beginning to: headstand signal after an unsuccessful hunt (n=23), wait without signalling after an unsuccessful hunt (n=74), hunt with a moray (n=82), be attended to at a cleaning station (n=100). The grouper’s signal is directed towards a referent We recorded 34 occurrences of the headstand signal by groupers ( Table 1 ), which followed 29 of 127 unsuccessful hunting episodes (four of which were followed by >1 headstanding event) in which prey escaped into a crevice. These headstands were performed by at least nine different grouper individuals during 187.25 h of focal observations of individual groupers in the wild. All headstands were performed directly over the location where the grouper ended an apparently unsuccessful hunt, as evidenced by the grouper making a high-speed burst that ended in a sudden stop, followed by the headstand signal over this location. Owing to the complex reef matrix, it was not possible to ascertain whether the prey fish remained at the location of its escape or moved to a different location unseen by the observer and probably also the grouper. Thus, the signal was used to indicate the location of the prey’s escape or the escaped prey itself. On five occasions one of the predators (twice a grouper, twice a moray, and once a wrasse) caught a fish during the ensuing joint attempt to reach the hidden prey. Table 1 A description of all 34 observed headstand signalling events. Full size table The grouper’s signal is mechanically ineffective We never observed a prey leaving its hiding place in response to the headstand signal itself; prey only abandoned cover after the arrival of a hunting partner capable of reaching into crevices (a moray or a wrasse). Also, if the headstand could be used directly to flush out or catch prey, groupers should perform headstanding in the absence of partners, but we never observed the signal in the absence of a potential recipient (see below). 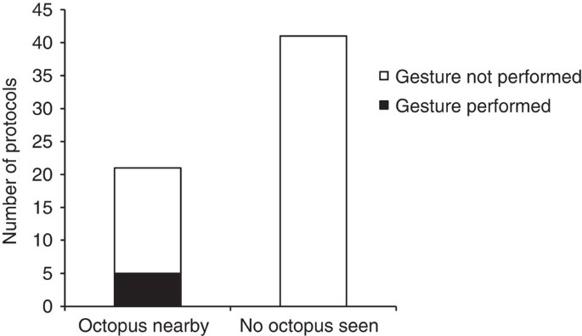Figure 2: The probability a headstand is performed by coral trout in the presence of an octopus. The number of focal follows of hunting coral trout in which the coral trout either did not perform or did perform a headstand gesture, seperated by whether an octopus was seen nearby (within 10 m) the coral trout at any stage during the protocol. The grouper’s signal is directed at a potential recipient A potential recipient was within the grouper’s visual range (hereafter ‘nearby'; see Methods) in all 34 cases where a grouper was observed to perform a headstand ( Table 2 ): in 14 cases a moray, 9 cases a wrasse, 10 cases a moray and wrasse and in 1 case a yellowlip emperor Lethrinus xanthochilus (hereafter ‘emperor’). These species were defined as potential recipients because they responded to the headstand signal by approaching the indicated location and could potentially flush out hidden prey. The term ‘potential recipient' acknowledges the fact that in cases where more than one potential recipient was nearby, we cannot be sure which organism was the intended recipient or received the signal (until it reacted to the signal). Table 2 Potential recipients nearby when the grouper began to signal. 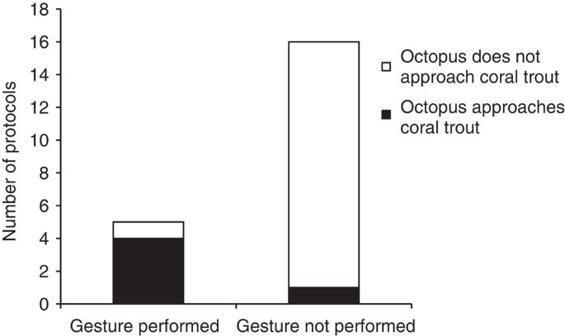Figure 3: Attraction of octopuses to headstanding versus non-signalling coral trout. The number of focal follows in which an octopus either does not approach or does approach a hunting coral trout, separated by whether the coral trout performed a headstand gesture or not. Full size table The grouper had been moving with a moray immediately before 7 of the 24 cases where a moray was nearby when the grouper performed a headstand, while in the other 17 cases the observer noted a moray sticking its head out of a crevice <10 m from the grouper ( Table 3 ). The grouper had been hunting with a wrasse immediately before 5 of the 19 cases where a wrasse was nearby when the grouper began to headstand signal. Four of these five events occurred after a wrasse inspecting the indicated crevice in response to a headstand began to swim off. On the other 14 occasions, it was evident the wrasse was nearby when signalling commenced due to it inspecting the indicated crevice within 1 min (and usually more quickly, but this temporal detail was not available. We term within 1 min as ‘immediately'). On the basis of swimming speed, it is unlikely the wrasse could have reached the grouper to inspect the indicated crevice this rapidly had it been outside the grouper’s visual range when signalling commenced (see Methods). On seven occasions the grouper waited for 2, 2, 3, 9, 10, 12 and 25 min over the location of a prey it had unsuccessfully hunted before beginning to headstand signal ( Table 4 ). For two of the seven delays a moray was within 10 m of the grouper (although it may not have initially been visible to the grouper), and for five delays no potential recipient was evident within 10 m of the grouper. A recipient arrived and inspected the indicated crevice immediately following six of the seven delayed headstands, suggesting that the grouper waited until a potential recipient swam by to perform the signal. Table 3 Methods to determine recipient nearby a signalling grouper. Full size table Table 4 Instances of delayed headstand signalling. Full size table Although a potential recipient was present for all 34 headstand signals, we needed to determine whether this could have occurred by chance. We did so using data on partner density and observed headstands from Mersa Bareika ( n =29), the main study site. At the study site (conservatively simplified to one dimension for analysis; see Methods) there was one moray per 100 m, meaning a 20% probability of one being <10 m (our association criterion) from a grouper by chance. A moray was observed <10 m from the grouper for 19 of the 29 headstand signals—significantly more than expected by chance (Binomial test: n =29, P <0.001). On average there was one wrasse per 350 m and the maximum distance a wrasse could feasibly see and reach a signalling grouper from immediately (within 1 min) was 26.4 m (see Methods), giving a 15% probability of one being within this range by chance. A wrasse was within this range for 16 of the 29 headstand signals as indicated by arriving to inspect the indicated crevice immediately or having been hunting with the grouper immediately before the signal—significantly more often than expected by chance (Binomial test: n =29, P <0.001). The grouper’s signal receives a voluntary response Morays freely became active in response to the headstand signal. Morays started to move in 14 of the 24 cases they were nearby a headstanding grouper, a significantly higher proportion than the 11 out of 38 cases described by Bshary et al . [19] in which morays started to move with a non-signalling grouper nearby (Fisher’s exact test: n =62, P =0.033). Wrasses were even more strongly attracted by the signal, investigating the indicated crevice immediately in all nine cases where they appeared to be the intended recipient of the signal (no moray or emperor was seen nearby the signalling grouper). Including events where a moray was also present, a grouper performing a headstand immediately after an unsuccessful hunt was joined by a wrasse (defined as coming within 10 m) that inspected the indicated crevice within 5 min in 12 out of 23 cases. This 12/23 probability is significantly higher than that of a wrasse joining a non-headstanding grouper within its first 5 min when waiting after an unsuccessful hunt (6/74 observations; Fisher’s exact test: n =97, P <0.001; Fig. 1 ), when hunting with a moray (2/82 observations; Fisher’s exact test: n =105, P <0.001), or when being inspected at a cleaning station (1/100 observations; Fisher’s exact test: n =123, P <0.001). Figure 1: Attraction of wrasses to the headstand gesture. The percentage of events in which a wrasse comes within 10 m of the grouper within 5 min of the grouper beginning to: headstand signal after an unsuccessful hunt ( n =23), wait without signalling after an unsuccessful hunt ( n =74), hunt with a moray ( n =82), be attended to at a cleaning station ( n =100). Full size image The grouper’s signalling has hallmarks of intentionality We provide evidence that the grouper’s headstand signal exhibits three features used as key indicators of an intentional signal production: persistence until the goal is reached, elaboration of the communication if it does not initially achieve its goal, and means-ends disassociation by using two signals for the same goal [20] , [21] , [22] . As evidence of persistence towards the apparent goal of the hunting partner flushing out the prey, groupers continued to perform the headstand signal until either a predator inspected the indicated crevice (27 cases), it became apparent the signal was not achieving its goal and an alternative signal was begun (6 cases), or the potential recipient did not respond (1 case). In the former 27 cases, the grouper stopped signalling as soon as the predator (moray, wrasse, or emperor) inspected the indicated crevice, requiring from mere seconds to a maximum of 7 min of signalling. Furthermore, on four of these occasions the grouper began to headstand signal as the wrasse it was inspecting a crevice with began to swim away, causing the wrasse to return on three occasions. The groupers’ response to ‘inappropriate’ behaviour by moray partners provides evidence for signal elaboration and means-end dissociation of the groupers’ communication. Morays often did not move to the location indicated by the grouper’s headstand. They failed to move on seven such hunts and moved in the wrong direction on four. The latter cases appear to be explained by morays following the reef formation, which may not guide them to the grouper’s location. In 9 out of 11 of these hunts where the moray did not inspect the headstand-indicated crevice, the grouper swam to within 20 cm of the moray (in three cases after a wrasse investigated the indicated crevice and then departed), performed the horizontal shimmy signal used for partner recruitment [19] , and then immediately swam back towards the previously indicated crevice. On four of these occasions the grouper sided with the moray and appeared to try and push it in the direction of the previously indicated crevice. The grouper was significantly more likely to elaborate on its headstand signal (by moving to the moray and shimmying) in response to a moray swimming away from its headstand signal (elaboration in 4/4 hunts) than a moray swimming towards its headstand (elaboration in 0/10 hunts) (Fisher’s exact test: n =14, P =0.001). Overall, groupers rarely succeeded in making the moray reach the crevice where the prey had hidden with their signal elaboration (1 out of 9 cases). Coral trout also perform the headstand signal The hunting relationship observed between coral trout and octopuses on the Great Barrier Reef appears to rely on the same complementary roles as the grouper’s partnership with morays and wrasses. The coral trout possesses speed to chase prey in the open and the octopus has long arms to access prey in crevices. The headstand gesture was observed on five occasions during a total of 62 follows of coral trout, averaging 50 min each. Only in three of these cases did the observer arrive before signalling began. In all three of these cases the coral trout had been associating closely with an octopus before signalling began, and the signal was conducted at the end of an apparently unsuccessful hunting strike by the coral trout that had taken it away from the octopus. The gesture was performed only when an octopus was nearby (within 10 m) the coral trout, and never during protocols where the coral trout made a hunting attempt but no octopus was observed nearby. Thus, the signal was significantly more likely to occur in hunting protocols where an octopus was seen nearby the coral trout (5 of 21 protocols) than protocols where an octopus was not seen (0 of 41 protocols; Fisher’s exact test: n =62, P =0.003; Fig. 2 ). Figure 2: The probability a headstand is performed by coral trout in the presence of an octopus. The number of focal follows of hunting coral trout in which the coral trout either did not perform or did perform a headstand gesture, seperated by whether an octopus was seen nearby (within 10 m) the coral trout at any stage during the protocol. Full size image On all but one occasion the octopus moved to the location indicated by the coral trout’s headstand, and octopuses were significantly more likely to approach a headstanding (4 of 5 protocols) than non-headstanding coral trout (1 of 16 protocols; Fisher’s exact test: n =21, P =0.004; Fig. 3 ). Figure 3: Attraction of octopuses to headstanding versus non-signalling coral trout. The number of focal follows in which an octopus either does not approach or does approach a hunting coral trout, separated by whether the coral trout performed a headstand gesture or not. Full size image Our results provide strong evidence that two species of fish, the grouper and coral trout, use referential gestures and that other fish species and an invertebrate respond to these signals appropriately. The signal draws attention to an object of interest to both the signaller and receiver, namely the hiding location of a prey fish, and appears to possess all five criteria derived from the attributes proposed by Pika and Bugnyar [13] to qualify as a referential gesture. Thus, the use of referential gestures is apparently not restricted to apes and a corvid. We suggest that the ability is perhaps not as rare as previously thought [13] : instead of being restricted to large-brained species the occurrence of referential gestures may be linked to ecological need [16] , [17] , [18] . Thus, further research may demonstrate the use of referential gestures by a wide range of vertebrate species including fishes. It has been suggested by Pika and Bugnyar [13] that the use of referential gestures by cooperative ravens strengthens the hypothesis of Vygotsky [23] that ‘evolutionary new inferential processes ensue when communication becomes governed by more cooperative motives’. Our demonstration of referential gestures by cooperatively hunting fishes appears to add further support to this argument, and cooperative interactions may provide a useful starting point in the search for referential gestures in other species. Other species that cooperate and for which signals have been described that may possess some if not all of the attributes of a referential gesture include domestic dogs [24] and captive dolphins [25] , which communicate about objects of interest with humans. Potential cases in the wild include bird species such as bowerbirds, green-backed sparrows, marabou storks and grass finches, which, in a manner similar to ravens, present non-food objects during pair formation and courtship [26] , [27] , [28] , [29] . Australian magpies perform a pointing-like action towards predators that may be used to indicate the danger to conspecifics [30] , although further research is required to exclude alternative explanations. Another potential example is the honeyguide, which leads humans to hidden beehives in a goal-orientated manner by making short flights in the hive’s direction, and then making a characteristic flight pattern over the location of the beehive [31] . The use of referential gestures has been interpreted as a cognitive feat in ravens [13] , and suggested to imply mental state attribution in chimpanzees [11] , which is the basis for a theory of mind [32] . The present study suggests that the attribution of such an advanced cognitive process to the use of referential gestures may be premature. As selection works on function rather than on mechanisms, different processes may underlie the same behavioural pattern in different taxa, but these have to be determined experimentally [16] , [33] . Our case study yields further support for the ecological approach to cognition, which emphasizes that the occurrence of cognitive solutions to specific problems is tightly linked to the specifics of a species’ ecology [16] , [17] , [18] . The occurrence of tool-use by termite hunting assassin bugs [34] , detour planning by jumping spiders [35] and symbolic language use by honey bees [36] offer further cases that should caution against the attribution of complex mental processes based on behavioural phenomena alone. The cognitive processes underlying the grouper and coral trout’s referential gestures are currently unknown. However, although fish have traditionally been considered relatively simple-minded, there is mounting evidence that their cognitive abilities are more advanced than previously thought [37] . In the present study, the observed ability of the grouper to wait above a hidden prey for up to 25 min before signalling to a passing predatory partner suggests it may perform at an ape-like level in a memory task commonly used to assess cognitive ability [38] . More generally, fishes may use complex social strategies in the context of intraspecific collaborative hunting [39] , social learning [40] , [41] and in cleaning interactions [42] , [43] , [44] , and demonstrate potentially complex cognitive processes such as transitive inference [45] and the ability to generalize [46] . On the neurophysiological level there is recent evidence that the reward structure of fish brains is similar to that of mammals [47] . In conclusion, primates and corvids do appear to be particularly cognitive clades, demonstrated by a variety of complex cognitive processes their constituent species are apparently capable of [14] , [15] . However, our results emphasize the importance of a more general evolutionary view of cognition [16] , [17] , [18] , which predicts that species evolve cognitive solutions according to their ecological needs. Data collection on groupers in the Red Sea Most observations were made between September 2002 and September 2004 in the eastern part of Mersa Bareika, Ras Mohammed National Park, Egypt. Along the 2,800 m coastline, 14 groupers, varying between 55 and 100 cm in total length (estimation), were recognized by individual spot patterns on their body. A snorkelling observer followed individual groupers continuously for up to 180 min for a total of 10,935 min of observation. Five additional observations were obtained during 300 min of focal follows at Shark Reef, Ras Mohammed National Park in September 2004. All relevant information was noted with a pencil on Plexiglas plates. Statistical analysis All statistical tests were non-parametric and performed in GraphPad QuickCalcs online software [48] . All reported P -values are two-tailed. Determining potential recipients nearby the grouper The visibility at the study site was typically 20–25 m for the human observer. As grouper vision appears to be adapted for distance given they frequently make hunting strikes on small individual prey fish up to 10 m away, we consider it likely that they could see at least as far as humans. Scoring the presence/absence of all potential hunting partners within visual range of the signalling grouper was not possible because of the visual limitations of a single snorkelling observer. The observer needed to constantly focus on the focal grouper, and combined with the tunnel-vision effect of the facemask this meant an approaching hunting partner would not usually be seen until it was <10 m from the grouper. This did not appear to be a substantial problem for morays as we never observed one being attracted to the grouper’s headstand from >10 m away, which should be well within the grouper’s visual range. We cannot exclude the possibility that the grouper saw morays that the observer did not. Wrasses presented a greater problem, as they are large (70 cm on average at the Mersa Bareika study site; Elodie Peingeon, unpublished data), deep-bodied fish that swim unconcealed in the open. They would thus be visible to the extent of the grouper’s mobile field of vision. Owing to the grouper being able to see a wrasse before the observer, we determined whether a wrasse was in visual range of a grouper that began to signal based on the arrival time of the wrasse. Wrasses moved at an average of 13.2 m min −1 relative to the coastline at the Mersa Bareika study site (Elodie Peingeon, unpublished data). On the basis of our observations, we estimate that they do not accelerate to more than twice this cruising speed to investigate a crevice indicated by a signalling grouper. Therefore, the maximum distance they could reach a signalling grouper from within 1 min is 26.4 m. This corresponds well to the 20–25 m visibility range, outside of which there should be no reason for a wrasse to accelerate from 13.2 m min −1 to reach a signalling grouper and hence reach it within 1 min. The same logic was used to classify an emperor as within the grouper’s visual range in the single case where an emperor investigated the crevice indicated by the grouper’s headstand signal. The null probability a grouper is nearby a partner species Almost all activity along the 2,800m long fringing reef study site occurred within a ∼ 50–100m wide band parallel to the coast. We can thus simplify the study site to one dimension (parallel to the coast), which gives a conservative overestimate of the probability a potential partner is nearby a signalling grouper. Both morays and wrasses have markings that allow individual identification, and these were used to identify all observed individuals within either a 700m representative section (morays) or the entire study site (wrasses), and hence calculate each species’ density. Data collection on coral trout on the Great Barrier Reef Observations were made between July 2010 and February 2012 at six sites around Lizard Island, the Great Barrier Reef, Australia. In most cases the snorkelling observer would follow an individual coral trout, noting relevant information on a Plexiglas plate. Opportunistic observations were also made when a coral trout was seen hunting with an octopus, and key behaviours were noted when the observer returned to shore. A coral trout was scored as ‘hunting’ if it made at least one high-speed hunting burst during the protocol. An octopus was defined as within visual range of the grouper if it was within 10 m of it. At this distance the human observer could see an octopus, and the coral trout’s vision is probably far better adapted to picking out objects at distance underwater given the long-distance (up to ∼ 10 m) hunting strikes it makes on small individual prey fish. How to cite this article: Vail, A. L. et al . Referential gestures in fish collaborative hunting. Nat. Commun. 4:1765 doi: 10.1038/ncomms2781 (2013).